Forbidden atomic transitions driven by an intensity-modulated laser trap Spectroscopy is an essential tool in understanding and manipulating quantum systems, such as atoms and molecules. The model describing spectroscopy includes the multipole-field interaction, which leads to established spectroscopic selection rules, and an interaction that is quadratic in the field, which is not often employed. However, spectroscopy using the quadratic (ponderomotive) interaction promises two significant advantages over spectroscopy using the multipole-field interaction: flexible transition rules and vastly improved spatial addressability of the quantum system. Here we demonstrate ponderomotive spectroscopy by using optical-lattice-trapped Rydberg atoms, pulsating the lattice light and driving a microwave atomic transition that would otherwise be forbidden by established spectroscopic selection rules. This ability to measure frequencies of previously inaccessible transitions makes possible improved determinations of atomic characteristics and constants underlying physics. The spatial resolution of ponderomotive spectroscopy is orders of magnitude better than the transition frequency would suggest, promising single-site addressability in dense particle arrays for quantum computing applications. Spectroscopy is a well-established, powerful tool in science for characterizing microscopic systems. Fields that use this tool range from precision metrology [1] (development of frequency standards [2] and high-precision sensing, such as gravitometry [3] ) to trace analysis [4] and chemical sensing [5] . Characterizing and manipulating particles using light is also the foundation of modern fields such as quantum optics [6] , computing [7] and information processing [8] , [9] . The interaction between a particle and a light field is described by the particle-field interaction Hamiltonian [10] , which includes a multipole-field interaction term and a ponderomotive (quadratic) interaction term. In the case of direct application of a radiation field to atoms, the dipole-field term typically dominates the total atom-field interaction and leads to the electric-dipole selection rules for atomic transitions. In contrast, the ponderomotive term may dominate the atom-field interaction when there is substantial spatial variation of the field intensity within the volume of the atom and when the intensity is modulated in time at a transition frequency of interest. In this case, any applicable selection rules are much less restrictive. To experimentally demonstrate an atomic transition via the ponderomotive interaction, we have chosen to use Rydberg atoms trapped in an intensity-modulated standing-wave optical lattice. Rydberg-atom optical lattices are an ideal tool for this demonstration because the atoms’ electronic probability distributions can extend over several wells of the optical lattice [11] , and Rydberg-Rydberg transitions are in the microwave regime [12] , a regime in which light-modulation technology exists. To further illuminate the use of such an intensity-modulated optical lattice for a demonstration of ponderomotive spectroscopy, we briefly examine the physics underlying the interaction between the Rydberg atom and the lattice light. The interaction between the atom and a light field is described by the following interaction Hamiltonian [10] : where p is the Rydberg electron’s momentum operator and A the vector potential of the light (the laser electric field E =−∂ A /∂ t ). The A · p term describes most types of atom-field interactions that are commonly engaged in spectroscopy [10] . These are classified as E1, M1, E2, etc. transitions, which follow well-established spectroscopic selection rules [13] . In the case of direct application of microwave radiation to Rydberg atoms, the electric-dipole (E1) selection rules apply (in first-order perturbation theory). In contrast, the quadratic A · A (ponderomotive) term allows us to drive transitions far beyond these selection rules by providing a substantial spatial variation of the field intensity within the volume of the atom and by modulating the intensity in time at the transition frequency between the coupled states. This method to drive atomic transitions is particularly effective in an amplitude-modulated optical lattice, as the lattice is spatially modulated with a period that is on the same scale as the Rydberg-atom diameter. In earlier work [14] , we proposed that, utilizing the A · A term, one can drive a wide variety of transitions beyond the usual spectroscopic selection rules. In this work, we report a successful demonstration of this spectroscopy. We trap 85 Rb atoms in a one-dimensional standing-wave optical lattice, formed by counter-propagating 1,064-nm laser beams. We drive the 58 S 1/2 →59 S 1/2 transition by sinusoidally modulating the lattice intensity at the resonant transition frequency, found to be 38.76861(1) GHz. The 58 S 1/2 →59 S 1/2 transition has been chosen because it is forbidden as a first-order electric-dipole (E1) transition, because its E2 coupling (due to the A · p term) is negligible and because for this transition we expect a high population transfer (due to the A · A term) in our intensity-modulated lattice [14] . Experiment In Fig. 1 we show a schematic of the experimental set-up. A continuous-wave (c.w.) 1,064-nm laser beam is split in a Mach-Zehnder interferometer (top) into a low-power and high-power beam. The low-power beam is sinusoidally modulated via an electro-optic fibre modulator driven by a tunable microwave-frequency voltage signal. This intensity-modulated low-power beam is coherently re-combined with the unmodulated high-power beam at the exit of the interferometer. In the atom-field interaction region (bottom), we form the standing-wave optical lattice by retro-reflecting the lattice beam. Cold 85 Rb Rydberg atoms are trapped with centre-of-mass positions near intensity minima of the lattice [11] (Methods). At these locations, the intensity modulation of the lattice results, via the A · A term, in a time-periodic atom-field interaction with a leading quadratic dependence on position (needed to couple states with an angular momentum change Δ l =0, 2 in first order). The proper combination of temporal and spatial intensity modulation is essential for utilizing the A · A term to realize the type of spectroscopy introduced in this report. 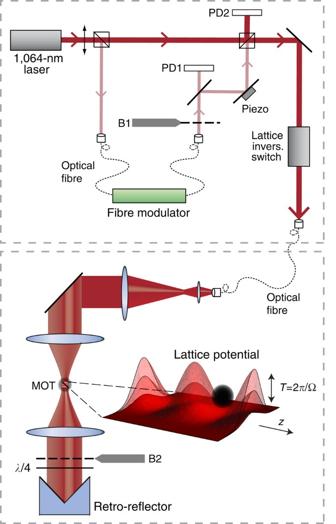Figure 1: Experimental set-up. A Mach-Zehnder interferometer (top) combines two 1,064-nm c.w. beams. One beam is intensity-modulated at frequency Ω by a fibre-based electro-optic modulator (‘Fibre modulator’), the operating point of which is set using photo-detector ‘PD1’. Using photo-detector ‘PD2’ and a piezo-electric transducer (‘Piezo’), the interferometer is locked such that the beams add up in phase. Rydberg atoms are laser-excited and optically trapped by lattice inversion. The optical lattice (bottom) is formed by retro-reflecting and focusing the 1,064-nm laser beam into the magneto-optical trap (‘MOT’). The lattice potential is intensity-modulated with periodT. Beam blocks (‘B1’,‘B2’) are used for signal interpretation. Details in Methods. Figure 1: Experimental set-up. A Mach-Zehnder interferometer (top) combines two 1,064-nm c.w. beams. One beam is intensity-modulated at frequency Ω by a fibre-based electro-optic modulator (‘Fibre modulator’), the operating point of which is set using photo-detector ‘PD1’. Using photo-detector ‘PD2’ and a piezo-electric transducer (‘Piezo’), the interferometer is locked such that the beams add up in phase. Rydberg atoms are laser-excited and optically trapped by lattice inversion. The optical lattice (bottom) is formed by retro-reflecting and focusing the 1,064-nm laser beam into the magneto-optical trap (‘MOT’). The lattice potential is intensity-modulated with period T . Beam blocks (‘B1’,‘B2’) are used for signal interpretation. Details in Methods. Full size image Spectroscopy signal In Fig. 2a we show the atomic transition 58 S 1/2 →59 S 1/2 driven via intensity modulation of the optical lattice. The 58 S 1/2 →59 S 1/2 spectrum is obtained by scanning the frequency of the microwave source driving the fibre modulator across the expected transition frequency. The spectral line shown in Fig. 2a is proof that the 58 S 1/2 →59 S 1/2 transition has been driven in a single step (in first order), at the fundamental transition frequency. The inset in Fig. 2a shows a simulated spectrum (details given in Supplementary Note 1 ). The simulation indicates that the sub-structure in the spectral line originates from different types of centre-of-mass trajectories of the atoms in the optical lattice. The dominant central peak results mainly from trapped atoms, whereas the small side structures result from atoms that traverse several lattice wells or that remain nearly stationary close to a lattice maximum during atom-field interaction [15] . The sub-structures, which are observed in the simulation, are not as clearly resolved in the experiment. This is most likely due to inhomogeneous broadening caused by optical-lattice imperfections. The simulation motivates us to fit the spectrum in Fig. 2a as a triple-Gaussian, which yields a central-peak location of 38.76861(1) GHz. 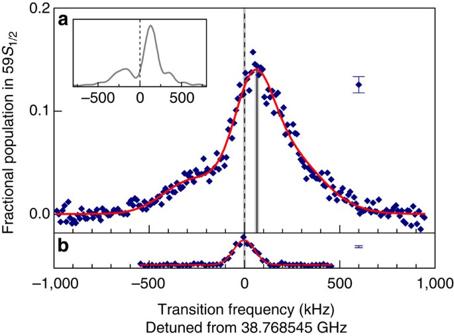Figure 2: The 58S1/2→59S1/2transition driven via intensity modulation of an optical lattice. The fraction of atoms in 59S1/2is shown. Spectral-line centres and background offset are determined by Gaussian fits (red curves). Grey areas represent s.e.m. of fit results for line centres. (a) Spectral line obtained by scanning the modulation frequency of the intensity-modulated optical lattice. The data are averages of 28 scans with 200 measurements each, taken under similar experimental conditions. Vertical error bar, s.e.m. of the 28 scans. Line centre is at 38.76861(1) GHz (black solid line). Inset, simulation results. (b) Reference scan performed by conventional two-photon microwave spectroscopy without the optical lattice, plotted versus twice the microwave frequency. The data are averages of 11 scans with 200 measurements each. Line centre is at 38.768545(5) GHz (black dashed line). Figure 2: The 58 S 1/2 →59 S 1/2 transition driven via intensity modulation of an optical lattice. The fraction of atoms in 59 S 1/2 is shown. Spectral-line centres and background offset are determined by Gaussian fits (red curves). Grey areas represent s.e.m. of fit results for line centres. ( a ) Spectral line obtained by scanning the modulation frequency of the intensity-modulated optical lattice. The data are averages of 28 scans with 200 measurements each, taken under similar experimental conditions. Vertical error bar, s.e.m. of the 28 scans. Line centre is at 38.76861(1) GHz (black solid line). Inset, simulation results. ( b ) Reference scan performed by conventional two-photon microwave spectroscopy without the optical lattice, plotted versus twice the microwave frequency. The data are averages of 11 scans with 200 measurements each. Line centre is at 38.768545(5) GHz (black dashed line). Full size image For reference, we have also driven the 58 S 1/2 →59 S 1/2 transition using direct application of microwave radiation at half the transition frequency; in this case, the transition results from a two-step (second-order) electric-dipole (E1) coupling through the 59 P 3/2 off-resonant intermediate state. In Fig. 2b we show the lattice-free 58 S 1/2 →59 S 1/2 spectral line, driven as a two-photon electric-dipole transition at half the transition frequency, using microwaves from a horn directed at the atom-field interaction region. This reference measurement yields a 58 S 1/2 →59 S 1/2 transition frequency of 38.768545(5) GHz. The transition frequencies measured in Fig. 2a,b are in good agreement with each other. The slight blue-detuning of the central peak in Fig. 2a relative to the peak in Fig. 2b is due to a light shift from the optical lattice. A calculation based on published quantum defect values [16] predicts a transition frequency at 38.7686(1) GHz, which is in agreement with the experimental measurements. We note that for the two-photon transition shown in Fig. 2b the microwave-induced AC Stark shift of the transition frequency is unusually small, due to near-cancellation of the upper- and lower-level AC shifts. We have estimated this shift of the transition frequency to be less than 500 Hz, which is insignificant in the above comparisons. Testing the nature of the atom-field interaction mechanism In Fig. 3 we show two tests that prove the spectral line shown in Fig. 2a is indeed caused by a perturbation due to the A · A atom-field interaction term in equation (1), which drives transitions via an intensity-modulated optical lattice. First, in Fig. 3a we verify that the transition does not originate from a combination of microwave leakage and stray DC fields. Although we carefully zero DC electric fields, a stray DC electric field in the atom-field interaction volume could, in principle, weakly perturb the 58 S 1/2 and 59 S 1/2 levels by adding some P -admixture to these levels. Any microwave-radiation leakage into the atom-field interaction region under the simultaneous presence of a DC electric field would drive the transition as an electric-dipole (E1) transition between the weakly perturbed 58 S 1/2 and 59 S 1/2 levels. To verify that our spectral line is not due to such a coincidence, we look for a spectral line while leaving all microwave equipment fully powered but blocking the weak, intensity-modulated optical beam in the Mach-Zehnder interferometer (beam block ‘B1’ in Fig. 1 ). In this case, the atoms are still trapped via the high-power, unmodulated beam. A stray DC electric field and leakage of microwave radiation into the chamber could then drive the transition as a single-step E1 transition. In Fig. 3a , we scan the microwave frequency in a manner identical to the procedure used for Fig. 2a . No spectral line is evident in Fig. 3a . This establishes that lattice light modulation, rather than microwave leakage in the presence of a stray DC electric field, drives the observed transition. 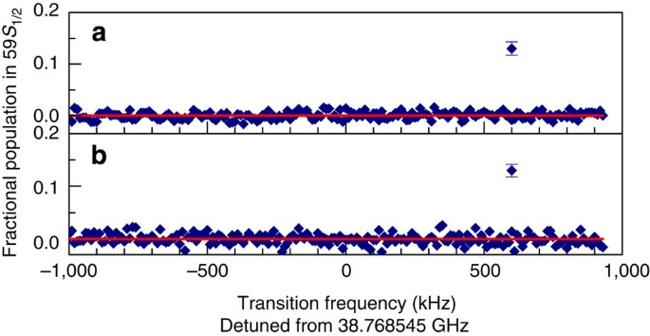Figure 3: Verification of the nature of the atom-field interaction mechanism. The fraction of atoms in 59S1/2is recorded as the modulation frequency is scanned. The absence of signals is important because it verifies the model presented in the text. Background offset is determined by a constant fit (red line). (a) Test to exclude dipole transitions caused by microwave leakage into the atom-field interaction region, performed using beam block ‘B1’ (Fig. 1) during frequency scans, while leaving the microwave source at full power. The data are averages of 16 scans with 200 measurements each. Error bar, s.e.m. of the 16 scans. (b) Test to exclude a stimulated electric-dipole Raman transition, performed using beam block ‘B2’ (Fig. 1) during frequency scans. The data are averages of 10 scans with 200 measurements each. Error bar, s.e.m. of the 10 scans. Figure 3: Verification of the nature of the atom-field interaction mechanism. The fraction of atoms in 59 S 1/2 is recorded as the modulation frequency is scanned. The absence of signals is important because it verifies the model presented in the text. Background offset is determined by a constant fit (red line). ( a ) Test to exclude dipole transitions caused by microwave leakage into the atom-field interaction region, performed using beam block ‘B1’ ( Fig. 1 ) during frequency scans, while leaving the microwave source at full power. The data are averages of 16 scans with 200 measurements each. Error bar, s.e.m. of the 16 scans. ( b ) Test to exclude a stimulated electric-dipole Raman transition, performed using beam block ‘B2’ ( Fig. 1 ) during frequency scans. The data are averages of 10 scans with 200 measurements each. Error bar, s.e.m. of the 10 scans. Full size image Next, we aim to distinguish between the A · A transition mechanism and a possible two-step A · p transition mechanism (equation (1)). As detailed in the next paragraph, either mechanism may, in principle, drive the observed 58 S 1/2 →59 S 1/2 transition via lattice modulation. However, these fundamentally distinct mechanisms differ in ways that can be tested experimentally. The modulated light field contains the frequency ω and frequency sidebands ω ±Ω, where ω is the light frequency, and Ω is the microwave modulation frequency of the light intensity (which is resonant with the 58 S 1/2 →59 S 1/2 transition). The presence of multiple frequencies allows, in principle, for the A · p term to couple 58 S 1/2 to 59 S 1/2 in a two-step (second-order) process via a stimulated Raman transition through one or more states that have an energy separation ≈ ℏ ω from the 58 S 1/2 and 59 S 1/2 levels. Following E1 selection rules, this mechanism would involve optical S → P and P → S electric-dipole transitions through distant intermediate P -states. The Raman coupling mechanism would be effective in both running-wave or standing-wave laser fields. In contrast, the coupling due to the A · A term is proportional to ‹59 S 1/2 | I ( z )|58 S 1/2 ›sin(Ω t ), where I ( z ) is the light intensity. For this coupling to be effective in first order, two conditions must be simultaneously fulfilled: the light intensity must substantially vary as a function of position z within the volume of the atom, and the modulation frequency Ω must correspond to the energy-level difference. Without spatial variation of I ( z ), the coupling vanishes due to the orthogonality of the atomic states. Hence, the A · A coupling is present in the intensity-modulated standing wave, while it is absent in an intensity-modulated running wave. To test whether it is a second-order A · p or a first-order A · A interaction that causes our spectroscopic signal, in Fig. 3b we exchange the intensity-modulated standing-wave optical lattice for an intensity-modulated running-wave beam by blocking the retro-reflected lattice beam with beam block ‘B2’ in Fig. 1 . We then scan the microwave frequency in a manner identical to the procedure used for Fig. 2a . No spectral line is evident in Fig. 3b . Therefore, the transition mechanism responsible for the spectral line observed in Fig. 2a is indeed a single-step atom-field interaction arising from the modulated optical standing-wave intensity (via a first-order A · A interaction), not a two-step electric-dipole Raman coupling process arising from the frequency sidebands in the light field (via a second-order A · p interaction). Dependence on experimental parameters Here we characterize the dependence of ponderomotive spectroscopy on several experimental parameters. In Fig. 4 we show the scaling behaviour of the spectral line width and amplitude on the atom-field interaction time. Experimentally, the interaction time t int is defined as the time between when the atoms are excited to the 58 S 1/2 state and when the atoms are ionized for detection (Methods), typically t int =6 μs. During the atom-field interaction time, the transitions are driven by the intensity-modulated lattice (which is always on), and the atoms undergo a square-pulse coupling to state 59 S 1/2 of duration t int . In the limit of weak saturation and assuming a Fourier-limited spectral profile of the driving field, the full-width-at-half maximum (FWHM) of the spectral line is expected to decrease with increased interaction time as ≈0.9/ t int . This agrees with the trend observed in Fig. 4 . A double-Gaussian fit of the 3-μs spectral line and triple-Gaussian fits of the 6-and-9-μs spectral lines (red solid curves in Fig. 4 ) indicate that the FWHM of the dominant Gaussian components in each line (red dashed curves) are within 20% of the Fourier limit. 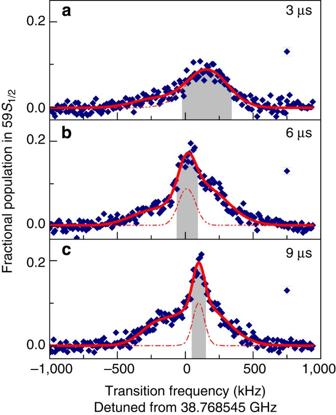Figure 4: Dependence of intensity-modulation-driven 58S1/2→59S1/2spectral line on interaction time. (a–c) For each interaction timetintwith the modulated lattice, the fraction of atoms in 59S1/2is recorded while scanning the microwave modulation frequency. The data are averages of 8 scans with 200 measurements each. Error bar, s.e.m. of the eight scans. The data fortint=3 (6 and 9) μs are fit with double- (triple-) peak Gaussians (red solid curves). The FWHM (grey areas) of the dominant Gaussians (red dashed curves) decreases with increasingtint, and the heights increase. Figure 4: Dependence of intensity-modulation-driven 58 S 1/2 →59 S 1/2 spectral line on interaction time. ( a – c ) For each interaction time t int with the modulated lattice, the fraction of atoms in 59 S 1/2 is recorded while scanning the microwave modulation frequency. The data are averages of 8 scans with 200 measurements each. Error bar, s.e.m. of the eight scans. The data for t int =3 (6 and 9) μs are fit with double- (triple-) peak Gaussians (red solid curves). The FWHM (grey areas) of the dominant Gaussians (red dashed curves) decreases with increasing t int , and the heights increase. Full size image Examining the spectral lines in Fig. 4 further, we also find that the maximum signal height approximately doubles between 3 and 6 μs; the additional increase between 6 and 9 μs is relatively minor. This observation is consistent with a Rabi frequency within the range of 50–100 kHz. This result is in qualitative agreement with our calculated Rabi frequency presented in Supplementary Note 2 . In Fig. 5 we summarize the dependence of the spectral-line height on additional experimental parameters. In Fig. 5a we investigate the dependence of spectral-line height on modulation strength, which is controlled by varying the amplitude of the microwave voltage signal V IM that drives the fibre modulator. As can be seen in equation (2), the Rabi frequency χ has a first-order Bessel function ( J 1 ) dependence on V IM . As the height of the spectral line indicates the peak fraction of population in 59 S 1/2 , we expect the height to scale as , for fixed t int and in the limit of weak saturation. In Fig. 5a , we plot the spectral line height as a function of the Bessel function argument, πV IM / V π , as we vary V IM . Fitting the data to a function proportional to yields good agreement. 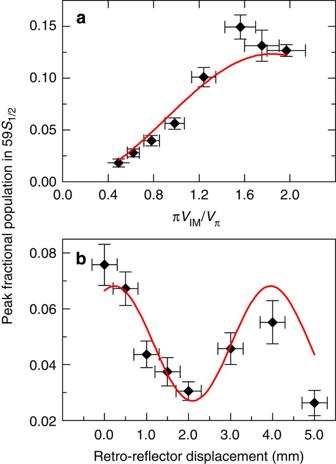Figure 5: Dependence of the height of the 58S1/2→59S1/2spectral line on experimental parameters. The peak fraction of 59S1/2atoms is recorded while varying experimental parameters. Each data point represents the observed peak height for an average of 5 (a) or 3 (b) scans with 200 measurements each. Vertical error bars, uncertainty of peak height. (a) Dependence onπVIM/Vπ, where we vary the microwave voltage amplitudeVIMapplied to the fibre modulator (Vπis fixed). Horizontal error bars are due to the uncertainty inVIM/Vπ. Red curve, fit proportional to. (b) Dependence on lattice retro-reflector distance from the atoms. Horizontal error bars, distance uncertainty. A sinusoidal curve (red) with a period of 4 mm is plotted for reference. Figure 5: Dependence of the height of the 58 S 1/2 →59 S 1/2 spectral line on experimental parameters. The peak fraction of 59 S 1/2 atoms is recorded while varying experimental parameters. Each data point represents the observed peak height for an average of 5 ( a ) or 3 ( b ) scans with 200 measurements each. Vertical error bars, uncertainty of peak height. ( a ) Dependence on πV IM / V π , where we vary the microwave voltage amplitude V IM applied to the fibre modulator ( V π is fixed). Horizontal error bars are due to the uncertainty in V IM / V π . Red curve, fit proportional to . ( b ) Dependence on lattice retro-reflector distance from the atoms. Horizontal error bars, distance uncertainty. A sinusoidal curve (red) with a period of 4 mm is plotted for reference. Full size image The spectral-line height also depends on the distance of the retro-reflector from the atoms. Both the incident and the retro-reflected intensity-modulated lattice beams can be viewed as periodic sequences of pulses with a repetition frequency Ω. The spectral-line height is maximal if the pulse trains of the incident and retro-reflected lattice beams arrive synchronously at the atoms’ location. Considering the time delay between the retro-reflected and incident pulses, it is seen that the spectral-line height should sinusoidally vary with the position of the retro-reflector mirror with a period of 4 mm. In Fig. 5b we plot the spectral-line height as a function of retro-reflector displacement over a range of a few millimetres. A sinusoidal curve with a period of 4 mm has also been plotted for reference. We observe good qualitative agreement, with deviations attributed to alignment drift of the excitation beams during acquisition of multiple data scans. This test provides another verification of our interpretation of the transition mechanism. In the analysis of our experimental evidence above, we have presented a classical-field picture. Spectroscopy using the ponderomotive interaction can also be interpreted using quantized fields. Using quantized fields, the lattice beams carry photons of three different frequencies: the optical carrier frequency, ω , and the optical carrier frequency with microwave sidebands, ω ±Ω. The transitions described in this work are due to absorption of a photon from one lattice beam and (simultaneous) re-emission of a photon into the other lattice beam, with the frequency difference between the two photons being Ω. It is necessary to have two counter-propagating (or non-co-propagating) fields to retain the spatial coupling between Rydberg levels. In the standard description of the interaction between an atom and a quantized electromagnetic field, the A · p term in equation (1) leads to well-known multipole transitions characterized as E1, M1, E2 and so on. The terms arise from an expansion of the exponential phase factor e ikz of the field, assuming a plane running wave propagating in the z -direction (without spatial amplitude modulation). The leading term of the expansion, E1, describes electric dipole transitions. These are often dominant, but higher-order terms such as the electric-quadrupole term, E2, are also used in precision spectroscopy [17] . All electromagnetic multipole transitions can, in principle, be driven in first order and are associated with well-known selection rules [10] . One common way to visualize first-order E1, M1, E2, etc., A · p transitions is via a three-branch Feynman diagram [10] (one vertex with three branches), in which an atom in an initial state transitions into a final state by absorption or emission of a photon. In contrast, the common way in which to visualize first-order A · A interactions is via a four-branch Feynman diagram [10] (one vertex with four branches), in which an atom in an initial state interacts simultaneously with an incoming and an outgoing photon, resulting in an atom in a final state. When a plane running wave is assumed, the atomic state and the photon energy are unchanged (in the non-relativistic case, relevant to this work). The process is an elastic scattering process that gives rise to Thomson scattering. Adding the second-order A · p interaction leads to the Kramers-Heisenberg formula, which describes Rayleigh scattering [10] , also an elastic scattering process. However, if the field amplitude substantially varies within the volume of the atom, as in the present work, then the field is not a plane running wave, and the atomic state and the photon energy may indeed be changed (an inelastic process). Such a state-changing A · A interaction is typically not considered in spectroscopy because the field intensity is typically constant within the volume of the atom. In our work we have demonstrated that a field inhomogeneity can be intentionally introduced into an atom-field system so that the A · A interaction results in state-changing transitions. Explicitly, since A · A is proportional to field intensity I , the matrix element ‹ R 2| A · A | R 1› representing a transition between two (different) Rydberg states | R 1› and | R 2› is different from zero only if ‹ R 2| I | R 1›≠0, that is, if the intensity I depends on position within the atom. For fixed intensity, the matrix element vanishes due to the orthogonality of the atomic states. Therefore, to drive transitions the light field must contain different spatial modes, to retain the spatial coupling between the Rydberg levels, and different optical frequencies, with a frequency difference corresponding to the energy difference between states | R 1› and | R 2›. An optical lattice that is amplitude-modulated at the desired atomic transition frequency, such as the lattice used in this work, satisfies these conditions. The transitions can be further described in terms of the four-branch Feynman diagram [10] referenced above: instantaneous exchange of a photon between two different field modes of the lattice yields different initial and final Rydberg states | R 1› and | R 2›. Finally, it should be noted that this process is not the same as stimulated Raman scattering because the latter is a second-order A · p process, which can be visualized by a sequence of two three-branch, A · p -type Feynman diagrams. Although transitions driven by the A · A term and electric-multipole transitions (E1, E2, E3, and so on, in first- and higher-order) may connect the same atomic states, we have explained above that the physical origins of these mechanisms are quite different. This results in different scaling laws. For instance, the Rabi frequencies of first-order multipole transitions scale proportional to the driving field, while Rabi frequencies in ponderomotive spectroscopy scale proportional to the intensity (see equation (2) below). One advantage of ponderomotive spectroscopy over established spectroscopic methods is flexible transition rules. Ponderomotive spectroscopy affords single-step access to atomic transitions that are forbidden by electric-dipole selection rules, an example of which is the 58 S 1/2 →59 S 1/2 transition demonstrated in this report. Atomic states with large differences in angular momentum can be coupled by choosing an appropriate atom size relative to the lattice period [14] . Accurate measurements of transitions for a wide range of angular-momentum separations may improve the determination of quantum defects and other atomic constants. As with any high-precision measurement method, light-induced level shifts must be considered. In spectroscopic studies of low-lying atomic states, E2 transitions in the optical spectral range between long-lived states can be driven as a single-photon process in low-intensity fields [17] . In contrast, in microwave spectroscopy of Rydberg levels, similar transitions are usually driven as E1 transitions in higher order (see, for instance, our Fig. 2b ), necessitating relatively strong microwave fields. These typically result in strong AC Stark shifts of the measured transition (the small shift seen in Fig. 2b is an anomoly of the specific transition in rubidium). In contrast, in ponderomotive spectroscopy light-induced shifts originate solely from the optical trapping fields acting on the Rydberg levels via the non-state-changing part of the A · A interaction. While in the present work these shifts are relatively large (on the order of 100 kHz), state-of-the-art laser cooling techniques will allow users to reduce the atom temperature from ~100 μK (our work) to ≲ 1 μK. This will allow a reduction of the trap depth and associated light shifts by at least a factor of 100. Furthermore, the differential light shift between selected upper and lower Rydberg levels cancels under certain ‘magic wavelength’ conditions, leading to at least one more order-of-magnitude reduction in the shift of the measured transition. We therefore believe that ponderomotive spectroscopy has immediate potential as a tool for high-precision spectroscopy of Rydberg atoms. Furthermore, another powerful innovation afforded by ponderomotive spectroscopy is a spatial resolution orders of magnitude better than the frequency of the transition would suggest. Electronic transitions in a particle are typically driven by applying radiation resonant with the transition frequency. The best possible spatial resolution will be at the diffraction limit of the applied radiation, which is on the order of the wavelength corresponding to the transition frequency and, in most cases, orders of magnitude larger than the particle size. In contrast, in ponderomotive spectroscopy, the frequency of the applied radiation is very different from the frequency of the transition being driven. The applied radiation is a standing wave with a wavelength on the order of the particle size. The frequency resonant with the desired transition is introduced by intensity-modulating the standing wave. In this report, a microwave-frequency atomic transition (typical resolution: centimetre-scale) has been driven by intensity-modulating a standing-wave optical lattice (typical resolution: micrometre-scale). This spatial addressability could streamline certain gate schemes in quantum computing, especially those schemes involving controlled electrostatic interactions between Rydberg atoms [7] , [8] . For example, by using site-selective transitions driven by ponderomotive spectroscopy, a recently proposed controlled- z gate scheme [18] could be modified such that the same Rydberg state is used for both control and target qubits (and no microwave field is needed). Ponderomotive spectroscopy may enable other advances in quantum computing, where single-site addressability plays a central role. In conclusion, we have successfully demonstrated ponderomotive spectroscopy. We have demonstrated major advantages over standard spectroscopy, including improved spatial addressability and flexible transition rules, which are relevant in a broad range of applications. Using a temporally and spatially modulated ponderomotive interaction, we have driven an atomic microwave transition forbidden by established electric-dipole selection rules, with a spatial resolution in the micrometre range. In our specific case, we have demonstrated ponderomotive spectroscopy using cold Rydberg atoms and an intensity-modulated standing-wave laser beam. One application of the method is in quantum computing [8] , [19] , where single-site addressability plays a central role. Another application is in precision measurement of atomic characteristics [20] and physical constants (for example, the Rydberg constant [21] , leading to the proton size [22] ); thereby, flexible spectroscopic transition rules will be very convenient. In the future, one may also explore the possibility of extending ponderomotive spectroscopy to smaller-sized atoms or molecules trapped in shorter-wavelength optical lattices. Preparation of cold Rydberg atoms in an optical lattice Initially, 85 Rb atoms are cooled to a temperature of about 150 μK in a magneto-optical trap (MOT). A one-dimensional, 1,064-nm optical lattice is applied to the MOT region. The optical lattice is formed by focusing an incident laser beam into the MOT region, retro-reflecting and re-focusing it. The incident beam interferes with the return beam and forms a standing wave. Pointing stability is greatly improved by using a retro-reflector rather than a plane mirror. See Fig. 1 in the main text for an illustration. The intensity ratio between the modulated and unmodulated portions of the incident lattice beam is about 1:100. The lattice has 880 mW of incident power at the MOT region with an 11-micrometre beam waist radius, and 490 mW of return power with a ~37-micrometre beam waist radius. See Supplementary Note 2 for a discussion of these numbers. Both MOT magnetic field and lattice light remain on throughout a data scan, while the MOT light is turned off during Rydberg atom excitation and probing. The Rydberg state is excited via a two-stage excitation 5 S 1/2 →5 P 3/2 →58 S 1/2 using 780-nm and 480-nm lasers, detuned from the intermediate 5 P 3/2 level by ≈1 GHz. Immediately after Rydberg-atom excitation, the lattice is inverted using an electro-optic component, required to efficiently trap Rydberg atoms at intensity minima. The Rydberg atoms are trapped in the optical field using the energy shift of the quasi-free Rydberg electron [11] . During a data scan, the Rydberg atom excitation laser wavelength is tuned so as to produce Rydberg atoms in the optical lattice at an average of 0.5 Rydberg atoms per experimental cycle. This ensures a negligible probability of atom–atom interactions. Zeroing the fields The electric field is zeroed before a series of data runs by performing Stark spectroscopy [23] of the 58 D 3/2 and 58 D 5/2 fine-structure levels, while scanning the potentials applied to a set of electric-field compensation electrodes. The residual field is <60 mV cm −1 . The MOT magnetic field, which is on during the experiment, does not cause Zeeman shifts of the 58 S 1/2 →59 S 1/2 transition. Lattice modulation While the 58 S 1/2 Rydberg atoms are trapped in optical lattice wells, the intensity of the lattice is modulated at the expected 58 S 1/2 →59 S 1/2 transition frequency. The electro-optic modulator used to perform the modulation is a fibre-coupled, polarization-maintaining, z -cut lithium niobate modulator, tunable from DC to 40 GHz. The modulator has an input optical power limit of 200 mW, which is, in the present experiment, insufficient for Rydberg-atom trapping. In a Mach-Zehnder-type interferometric set-up, we split the 1,064-nm laser into a high-power (3.9 W), unmodulated beam and a low-power (190 mW), intensity-modulated beam, which is passed through the fibre modulator. The two beams are coherently re-combined at the exit beam-splitter of the Mach-Zehnder interferometer. The re-combined beam incident at the MOT region has ~1 W of average power, which is sufficient for Rydberg atom trapping. See Supplementary Note 2 . Operating point of the fibre modulator The fibre modulator has two voltage inputs, one for the microwave voltage signal and another for a DC bias voltage. As described by equations (1 and 2) in Supplementary Note 2 , the intensity transmitted through the fibre modulator depends on the values of these voltage inputs. For most of the work, the amplitude of the microwave signal is set to V IM = V π /2, which yields maximal intensity modulation when the DC bias voltage is set for a time-averaged transmission through the modulator that equals 50% of the maximum possible. Owing to thermal drifts in the fibre modulator, the DC bias voltage must be actively regulated to maintain this operating point. The lock circuit utilizes a photo-detector (‘PD1’ in Fig. 1 ) and a PID regulator. Locking the interferometer Owing to drifts in the optical path length difference between the arms of the Mach-Zehnder interferometer, the path length of one of the interferometer arms must be actively regulated to maintain a fixed phase difference at the recombination beam-splitter. This phase difference is locked so that the intensity sent to the experiment is at a maximum (by maintaining an intensity minimum at the unused output of the recombination beam-splitter). The lock circuit utilizes a photo-detector (‘PD2’ in Fig. 1 ), a mirror mounted on a piezo-electric transducer (‘Piezo’ in Fig. 1 ), and a PID regulator. Rabi frequency estimate To initialize certain experimental parameters (such as atom-field interaction time), we must make an estimate of the expected Rabi frequency. Because of the coherent mixing of the low-power, modulated lattice beam with a high-power, unmodulated beam, the time-averaged lattice depth is large enough that most atoms remain trapped in the lattice while the 58 S 1/2 →59 S 1/2 transition is probed. The coherent mixing of the two beams provides the additional benefit that it enhances the modulation in the atom-field interaction region, resulting in a much larger 58 S 1/2 →59 S 1/2 coupling than would be possible with the weak modulated beam alone. The Rabi frequency for a transition | n , l , m ›→| n′ , l′ , m′ › between two Rydberg states that are resonantly coupled by the intensity-modulated lattice is where V IM is the amplitude of the microwave voltage signal that drives the fibre modulator, V π is the voltage difference between minimum and maximum intensity transmission through the modulator (a fixed modulator property), ε is the intensity ratio at the atom location between the return and incident beams forming the lattice, e is electron charge, m e is electron mass, ω is the angular frequency of the optical-lattice light, and and are the incident intensities of the modulated and unmodulated lattice beams at the atom location, respectively. The transition matrix element (unitless) has been derived in previous work [14] and is 0.215 for the 58 S 1/2 →59 S 1/2 transition for an atom located at a minimum in our lattice. This value is large compared with those of other possible transitions due to a favourable ratio between atom size and lattice period (which is on the order of one). A detailed derivation of equation (2) is given in Supplementary Note 2 along with values for the parameters listed above, yielding a typical Rabi frequency estimate on the order of 100 kHz. The in-phase addition of the fields corresponding to intensities and , using the Mach-Zehnder beam combination set-up, leads to the enhancement term in square brackets in equation (2). In our experiment, the Rabi frequency is enhanced by a factor of ≈20, which aids significantly in observing the transition. While in our experiment the enhancement afforded by the interferometric set-up is critical for a successful demonstration, different laser wavelengths, modulation schemes, sub-Doppler and evaporative cooling techniques or the use of separate trapping and modulation beams could make the interferometric set-up unnecessary. Detection The spectral line is detected through state-selective field ionization [12] , in which Rydberg atoms are ionized by a ramped electric field. Freed electrons are detected by a micro-channel plate, and detections on the micro-channel plate are registered by a pulse counter. Counting gates are synchronized with the field ionization ramp to enable state-selective detection of the 58 S 1/2 and 59 S 1/2 Rydberg levels. Read-out protocol During a data scan, the microwave frequency of the intensity-modulation is stepped across the expected 58 S 1/2 →59 S 1/2 resonance frequency. At each microwave frequency step, the pulse counter registers counts for 200 experimental cycles. Average counts per cycle are recorded before advancing to the next frequency step. The interferometer lock status is queried before and after each set of 200 experimental cycles. If either query indicates an unlocked interferometer, the data for that frequency step are ignored and re-taken. How to cite this article: Moore, K. R. et al . Forbidden atomic transitions driven by an intensity-modulated laser trap. Nat. Commun. 6:6090 doi: 10.1038/ncomms7090 (2015).